In vivoconversion of astrocytes to neurons in the injured adult spinal cord Spinal cord injury (SCI) leads to irreversible neuronal loss and glial scar formation, which ultimately result in persistent neurological dysfunction. Cellular regeneration could be an ideal approach to replenish the lost cells and repair the damage. However, the adult spinal cord has limited ability to produce new neurons. Here we show that resident astrocytes can be converted to doublecortin (DCX)-positive neuroblasts by a single transcription factor, SOX2, in the injured adult spinal cord. Importantly, these induced neuroblasts can mature into synapse-forming neurons in vivo . Neuronal maturation is further promoted by treatment with a histone deacetylase inhibitor, valproic acid (VPA). The results of this study indicate that in situ reprogramming of endogenous astrocytes to neurons might be a potential strategy for cellular regeneration after SCI. Injury to the spinal cord leads to irreversible loss of neurons and the disruption of ascending and descending spinal tracts with consequent impairments of motor and sensory function below the injury [1] , [2] . Unlike certain regions in the adult brain where neurogenesis persists [3] , the spinal cord lacks the ability to produce new neurons in adulthood [4] , [5] , [6] . A key challenge is how to restore neurons after spinal cord injury (SCI). Cell transplantation using stem or differentiated cells has attracted the most attention as a potential therapeutic strategy for SCI [7] . The establishment of induced pluripotent stem cells (iPSCs) [8] from a patient’s somatic cells resolves the ethical controversies and immunological rejection, which are problems associated with cells derived from human fetal tissues. Recent studies also showed that grafted fetal or iPSC-derived neural stem cells (NSCs) can overcome an inhibitory environment to achieve neuronal growth and form a functional relay, thus promoting spinal cord repair [9] , [10] . These results clearly demonstrate that neural networks in the adult spinal cord exhibit structural plasticity, which provides a strong rationale for cell-based therapy. However, transplantation-based cell therapy faces several major hurdles for treating SCI in human patients. First, the time required to prepare cells for autologous transplantation is longer than the therapeutically optimal time window. Extensive studies showed that cells transplanted in the subacute phase, but not the chronic phase, could have functional improvement [11] , [12] . However, derivation and characterization of iPSCs from patient somatic cells is a very time-consuming process. This is further exacerbated because these pluripotent cells need to be extensively expanded and differentiated in culture before transplantation [13] . Second, there is potential for tumour formation from residual undifferentiated stem cells in the injured environment [14] . Third, the transplantation procedure induces secondary injury to the spinal cord. A relatively large quantity of cells is frequently needed for transplantation, which can result in unintended damage to preexisting functional neural circuits, fluid leak and the formation of cystic tissue at the injection site(s). Continued refinement of cell transplantation is required to overcome these major hurdles. As an alternative to transplantation, we examined the possibility of reprogramming endogenous non-neuronal cells, such as scar-forming astrocytes, into neurons in the adult spinal cord. This approach is based on recent progress in the reprogramming field. In cell culture, the fates of many somatic cells can be re-specified by the forced expression of a few transcription factors [8] , [15] , [16] , [17] , [18] . Most importantly, adult pancreatic exocrine cells in vivo can be directly transformed into insulin-secreting β-cells by three transcription factors [19] . Cardiac fibroblasts in injured adult mouse heart could be reprogrammed to cardiomyocytes by three or four factors [20] , [21] . Recent studies also showed the potential of converting brain astrocytes directly to neurons by the forced expression of neurogenic factors [22] , [23] . These findings raise the possibility that endogenous non-neuronal cells, such as astrocytes, could be reprogrammed in vivo to neurons in the adult spinal cord. Astrocytes are broadly distributed throughout the spinal cord [24] . After SCI, astrocytes proliferate to form a scar that preserves the integrity of surrounding cells. However, the persistence of a glial scar is detrimental to functional recovery of a damaged spinal cord, largely because this scar not only forms a physical barrier but also secretes inhibitors of axonal growth [25] . Interestingly, astrocytes are amenable to reprogramming in culture [17] , [26] , [27] , [28] and in the adult brain [22] , [23] . Our recent studies also showed that brain astrocytes can be converted to induced adult neuroblasts [29] . Because of regional heterogeneity of astrocytes, however, it is unclear whether the fate of astrocytes in the adult spinal cord can be reprogrammed in vivo . In this study, we screened for factors that could induce neurogenesis in the adult spinal cord and found that ectopic SOX2 is sufficient to convert endogenous spinal astrocytes to proliferative DCX-positive neuroblasts, which eventually generate mature neurons. Neuronal survival and maturation are further enhanced by treating the mice with valproic acid (VPA). Our study indicates that resident astrocytes in the injured adult spinal cord can be manipulated to produce neurons by defined factors, raising the possibility of using these cells as a source for in situ repair of SCI. Inducing neurogenesis in the adult spinal cord We used a lentiviral gene delivery system to target both proliferating and quiescent cells in the adult mouse spinal cord. Gene expression was regulated by the human glial fibrillary acidic protein ( hGFAP ) promoter, which is active primarily in astrocytes [30] . To further examine the cell types targeted by this lentiviral system in the adult spinal cord, 1.5 μl of green fluorescent protein ( GFP )-expressing virus ( hGFAP - GFP ) was injected at two positions 3–5 mm apart at the thoracic level 8 (T8). One week post viral injection (wpi), immunohistochemical analyses of longitudinal sections around the injected regions showed that GFP + cells were detectable in a broad area, especially in the white matter, reaching a distance of ~3.0 mm from the injection site both rostrally and caudally ( Supplementary Fig. 1a ). While a few GFP + cells were stained positive for markers of neurons (NeuN, <0.82%), oligodendrocyte precursors and pericytes (OLIG2, 4.94±3.10% and NG2, 4.36±2.83%; mean±s.d., n =3), the vast majority expressed the astrocyte-specific marker GFAP (95.09±4.15%, mean±s.d., n =3) ( Supplementary Fig. 1b–e,i ). Markers for mature oligodendrocytes (MBP and PLP) or microglia (IBA1) were not detected in GFP + cells ( Supplementary Fig. 1f–i ). These results indicate that spinal astrocytes are the major cell type targeted by lentivirus under the regulation of hGFAP promoter. On the basis of their roles in NSCs and/or neurogenesis, 12 genes ( SOX2 , PAX6 , NKX6.1 , NGN2 , ASCL1 , OLIG2 , SOX11 , Tlx , OCT4 , c-MYC , KLF4 and PTF1a ) were chosen as candidates. Lentivirus expressing these candidates under the hGFAP promoter was individually injected into the T8 region of the adult spinal cord and analysed for their ability to induce adult neurogenesis ( Fig. 1a ). Neurogenesis was initially examined by staining for the expression of doublecortin (DCX), a microtubule-associated protein that is broadly expressed in neuroblasts and immature neurons during development and in neurogenic regions of the adult brain [31] , [32] . DCX expression is mainly associated with adult neurogenesis but not with reactive gliosis or regenerative axonal growth [33] . Consistent with these results, DCX was not detected in either intact spinal cords or those with hemisection-induced injuries ( Supplementary Fig. 2 ). In sharp contrast, DCX + cells were identified in spinal cords injected with virus expressing SOX2 but none of the other 11 candidate genes at 4 wpi. This was further confirmed with a virus expressing GFP-T2A-SOX2 so that virus-transduced cells could be identified by the coexpression of GFP ( Fig. 1b–d ). 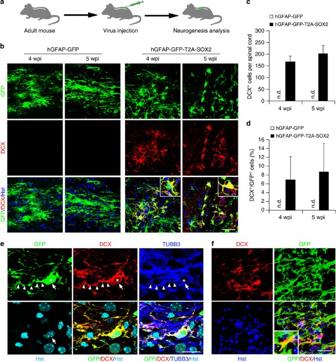Figure 1: Induction of DCX+cells in the adult mouse spinal cord. (a) Experimental scheme. (b) DCX+cells are detected in animals injected with lentivirus expressing SOX2 but not control GFP at 4 or 5 wpi. Nuclei were counterstained with Hoechst 33342 (Hst) (c,d) Quantification of SOX2-induced DCX+cells around the virus-injected regions in adult spinal cords (mean+s.d.;n=3 mice per group; n.d., not detected). (e) Confocal images of a representative DCX+cell (indicated by arrows). SOX2-induced DCX+cells are traced by the coexpressed GFP, indicating an origin of virus-infected cells. They are also co-labelled by TUBB3 and have bipolar or multipolar processes. Asterisks and arrowheads indicate cell bodies and neuronal processes, respectively. (f) Representative images of DCX+cells induced in the spinal cord of aged mice (>12 months). Scale bars, 50 μm (b,f) and 20 μm (e). Figure 1: Induction of DCX + cells in the adult mouse spinal cord. ( a ) Experimental scheme. ( b ) DCX + cells are detected in animals injected with lentivirus expressing SOX2 but not control GFP at 4 or 5 wpi. Nuclei were counterstained with Hoechst 33342 (Hst) ( c , d ) Quantification of SOX2-induced DCX + cells around the virus-injected regions in adult spinal cords (mean+s.d. ; n =3 mice per group; n.d., not detected). ( e ) Confocal images of a representative DCX + cell (indicated by arrows). SOX2-induced DCX + cells are traced by the coexpressed GFP, indicating an origin of virus-infected cells. They are also co-labelled by TUBB3 and have bipolar or multipolar processes. Asterisks and arrowheads indicate cell bodies and neuronal processes, respectively. ( f ) Representative images of DCX + cells induced in the spinal cord of aged mice (>12 months). Scale bars, 50 μm ( b , f ) and 20 μm ( e ). Full size image SOX2-induced DCX + cells were mainly identified surrounding the virus-injected region and showed typical immature neuronal morphology with bipolar or multipolar processes ( Fig. 1b,e ). They coexpressed betaIII-tubulin (TUBB3, also known as TUJ1), a pan-neuronal marker, and were labelled by GFP, showing an origin of virus-transduced cells ( Fig. 1e ). The induction efficiency of DCX + cells was estimated at 6–8% of GFP + cells surrounding the core injection sites at 4 or 5 wpi ( Fig. 1d ). Interestingly, ectopic SOX2 also resulted in the production of DCX + cells in aged mice (>12 month, Fig. 1f ). Together, these data suggest that neurogenesis can be induced by a single transcription factor, SOX2, in the adult spinal cord, similar to observations made in the adult striatum [29] . Inducing neurogenesis in spinal cords with severe injuries Severe traumatic injury to the adult spinal cord causes massive cell death, inflammation and gliosis [1] , [25] , [34] , which result in a pathological microenvironment drastically different from that of the needle injection-induced stab wound injury. To examine whether neurogenesis could also be induced under this clinically-relevant pathological condition, we injected lentivirus into the parenchyma of severely injured spinal cord immediately after hemisection at the T8 level ( Fig. 2a ). The two injection sites were 1.5 mm away from the injury core on each side ( Supplementary Fig. 3a ). Histological analyses were performed on spinal cord sections spanning the lesion site. Similar to what was observed in the intact spinal cord, the control virus hGFAP - GFP could efficiently transduce cells surrounding the injection sites with a majority expressing the astrocyte marker GFAP (95.21±3.95%, mean±s.d., n =3; Supplementary Fig. 3b,i ). Only a small percentage of GFP + cells expressed markers for neurons, oligodendrocyte precursors or pericytes (NeuN + , <0.91%; OLIG2, 4.73±2.94%; NG2, 3.73±2.74%; mean±s.d., n =3) ( Supplementary Fig. 3c–e,i ). None expressed the markers for mature oligodendrocytes MBP and PLP or the microglia marker IBA1 ( Supplementary Fig. 3f–i ). These results are very similar to those in spinal cords without the hemisection ( Supplementary Fig. 1 ), suggesting that severe injury does not change the cell types targeted by lentivirus. 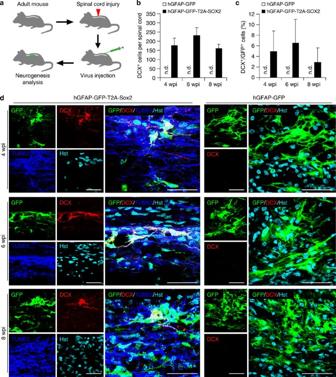Figure 2: Inducing neurogenesis in the adult spinal cord after severe injury. (a) Experimental scheme. Lentivirus was injected into the spinal cord immediately after hemisection at the T8 level. (b) Quantification of SOX2-induced DCX+cells around the virus-injected regions in injured spinal cords (mean+s.d.;n=4 mice per group; n.d., not detected). (c) Percentage of GFP+cells expressing DCX around the virus-injected regions in injured spinal cords (mean+s.d.;n=4 mice per group; n.d., not detected). (d) Representative images of DCX+cells induced by virus expressing SOX2 but not the GFP control at 4, 6 or 8 wpi. Scale bar, 40 μm. Figure 2: Inducing neurogenesis in the adult spinal cord after severe injury. ( a ) Experimental scheme. Lentivirus was injected into the spinal cord immediately after hemisection at the T8 level. ( b ) Quantification of SOX2-induced DCX + cells around the virus-injected regions in injured spinal cords (mean+s.d. ; n =4 mice per group; n.d., not detected). ( c ) Percentage of GFP + cells expressing DCX around the virus-injected regions in injured spinal cords (mean+s.d. ; n =4 mice per group; n.d., not detected). ( d ) Representative images of DCX + cells induced by virus expressing SOX2 but not the GFP control at 4, 6 or 8 wpi. Scale bar, 40 μm. Full size image No DCX + cells were detected in the injured spinal cords injected with the control virus hGFAP - GFP at 4, 6 or 8 wpi ( Fig. 2b–d ). In stark contrast, these cells were specifically induced by the injection of hGFAP-GFP-T2A-SOX2 virus ( Fig. 2b–d ). All the induced DCX + cells also expressed GFP indicating an origin from virus-transduced cells ( Fig. 2d ). An estimation of 3–6% of GFP + cells surrounding the core viral injection sites were reprogrammed by SOX2 to become DCX + cells between 4–8 wpi ( Fig. 2c ). These DCX + cells also stained positive for the neuronal marker TUBB3 ( Fig. 2d ). Together, these data indicate that neurogenesis can be induced by SOX2 in an injured environment of the adult spinal cord. SOX2-induced neurogenesis originates from spinal astrocytes The cellular source for SOX2-induced DCX + cells was determined by genetic lineage tracing. Gene expression under the hGFAP promoter was not detected in mature oligodendrocytes or microglia ( Supplementary Figs 1,3 ), thus excluding them as a possible origin for SOX2-induced DCX + cells. Although less than 5% of NG2 + cells were targeted by the hGFAP promoter ( Supplementary Figs 1,3 ), these cells were specifically examined as they are cycling precursors for oligodendrocytes, exhibit plasticity after injury in the adult central nervous system [35] and are amenable to fate reprogramming in culture [15] . NG2 + cells and their derivatives were traced using Ng2-Cre BAC transgenic mice [36] and the reporter Rosa-YFP ( Fig. 3a ). A respective 71 and 64% of YFP + cells expressed NG2 and OLIG2 in the adult spinal cord ( Supplementary Fig. 4a,b,d ). Markers for astrocytes (GFAP), microglia (IBA1) or neurons (TUBB3) were not detected in YFP-traced cells ( Supplementary Fig. 4c,d ). Transgenic mice were then injected with hGFAP-SOX2 lentivirus and examined at 5 wpi. Immunohistochemistry showed that DCX + cells were induced around the virus-injected regions but none co-labelled with YFP ( Fig. 3b ). This result indicates that DCX + cells induced by SOX2 under the hGFAP promoter do not originate from NG2 + cells in the adult spinal cord. 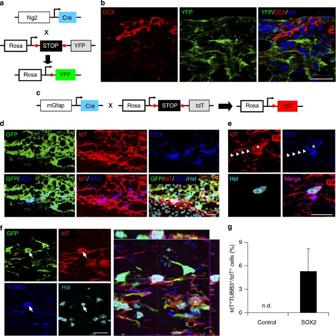Figure 3: SOX2-induced new neurons originate from spinal astrocytes. (a,b) SOX2-induced DCX+cells do not come from NG2+cells.Ng2-Cre;Rosa-YFPmice (a) were injected with SOX2-expressing or empty lentivirus and were analysed at 5 wpi. Confocal images are shown in panel (b). (c–g) SOX2-induced new neurons originate from astrocytes. (c)mGfap-Cre;Rosa-tdTmice were injected with virus expressing either GFP-T2A-SOX2 or GFP (as a control) and were analysed at 5 wpi. (d) Representative confocal images showing that SOX2-induced DCX+cells originate from lentivirus-infected astrocytes (indicated by GFP+tdT+). (e) Higher magnification views of a tdT-labelled DCX+cell. Asterisks and arrowheads indicate cell bodies and processes, respectively. (f,g) SOX2-induced TUBB3+neurons are derived from virus-infected astrocytes (indicated by GFP+tdT+). Traced neurons were quantified in virus-injected regions (mean+s.d.;n=5 mice per group; n.d., not detected). Scale bar, 20 μm (b,d–f). Figure 3: SOX2-induced new neurons originate from spinal astrocytes. ( a , b ) SOX2-induced DCX + cells do not come from NG2 + cells. Ng2-Cre;Rosa-YFP mice ( a ) were injected with SOX2-expressing or empty lentivirus and were analysed at 5 wpi. Confocal images are shown in panel ( b ). ( c – g ) SOX2-induced new neurons originate from astrocytes. ( c ) mGfap-Cre;Rosa-tdT mice were injected with virus expressing either GFP-T2A-SOX2 or GFP (as a control) and were analysed at 5 wpi. ( d ) Representative confocal images showing that SOX2-induced DCX + cells originate from lentivirus-infected astrocytes (indicated by GFP + tdT + ). ( e ) Higher magnification views of a tdT-labelled DCX + cell. Asterisks and arrowheads indicate cell bodies and processes, respectively. ( f , g ) SOX2-induced TUBB3 + neurons are derived from virus-infected astrocytes (indicated by GFP + tdT + ). Traced neurons were quantified in virus-injected regions (mean+s.d. ; n =5 mice per group; n.d., not detected). Scale bar, 20 μm ( b , d – f ). Full size image In contrast, astrocytes are the most likely cellular origin for the induced neurons since they are the predominant cell type targeted by lentivirus under the hGFAP promoter ( Supplementary Figs 1,3 ). This hypothesis was examined by genetic lineage tracing using the transgenic mGfap-Cre line 77.6 , which was reported to exclusively trace astrocytes in the forebrain [23] . We crossed this line to Rosa-tdTomato ( tdT ) reporter [37] and examined the identity of the labelled cells in the adult spinal cord ( Fig. 3c , Supplementary Fig. 5 ). On the basis of GFAP expression, 71.32±6.75% of astrocytes were labelled by the reporter tdT. Among tdT + cells, the vast majority expressed the astrocyte markers GFAP (97.36±3.24%, mean±s.d., n =3) and glutamine synthetase (GS, 95.14±3.86%, mean±s.d., n =3), while fewer than 5% were positive for NG2 or OLIG2 ( Supplementary Fig. 5a–d,f ). Markers for microglia (IBA1 + ) or neurons (NeuN + , MAP2 + and TUBB3 + ) were not expressed in traced cells ( Supplementary Fig. 5e,f ). Adult mGfap-Cre;Rosa-tdT mice were then injected with lentivirus expressing either GFP (as a control) or GFP-T2A-SOX2 and examined at 5 wpi. Immunohistochemistry showed that ectopic SOX2 induced DCX expression in tdT + cells ( Fig. 3d ). Importantly, a fraction of the traced cells were also labelled by the neuronal marker TUBB3 (~5%) in the core spinal regions injected with SOX2 virus ( Fig. 3f,g ). In stark contrast, these neuronal markers were not detectable in tdT-traced cells in spinal cords injected with the control virus ( Fig. 3g ), although GFP expression showed a clear infection of these cells ( Supplementary Fig. 6 ). These results indicate that SOX2-induced new neurons come from resident astrocytes. Cell transplantation assays were performed to further confirm these results. Spinal astrocytes were isolated from neonatal mGfap-Cre;Rosa-tdT mice, cultured for 7–10 days in serum-containing medium, and subsequently passaged once. tdT + astrocytes were then purified by fluorescence-activated cell sorting and infected with either hGFAP - GFP or hGFAP-GFP-T2A-SOX2 lentivirus ( Fig. 4a ). The astrocytic identity and expression of ectopic GFP and SOX2 were confirmed by immunocytochemistry ( Fig. 4b,c ). Three days post viral infection (dpi), these cells were transplanted into the spinal cords of adult immunodeficient NOD scid gamma (NSG) mice. When examined at 4 wpi, none of the control GFP virus-infected tdT + cells stained positive for the neuronal marker TUBB3 ( Fig. 4d ). In contrast, TUBB3 expression was clearly detectable in tdT + cells that were infected with the hGFAP-GFP-T2A-SOX2 virus before transplantation ( Fig. 4d ). GFP expression in the latter group was also downregulated, reflecting much reduced activities of the hGFAP promoter in converted cells. By 5 wpi, some of the tdT + cells in the SOX2 group started to express MAP2, a marker for mature neurons. These results demonstrate that the ectopic expression of SOX2 can convert transplanted spinal astrocytes to neurons in the adult spinal cord. 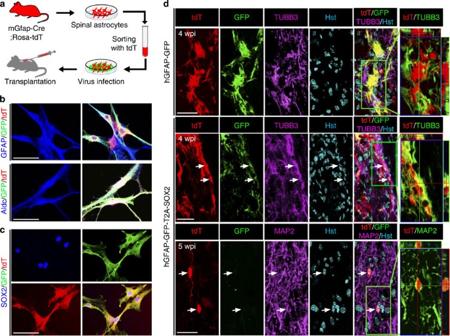Figure 4:In vivoconversion of engrafted astrocytes to neurons. (a) Experimental scheme. Spinal astrocytes cultured frommGfap-Cre;Rosa-tdTmice were purified based on tdT expression. Three dpi, cells were infected with lentivirus and transplanted into the spinal cord of NSG mouse. (b) Immunocytochemistry showing the expression of GFAP and Aldolase c (Aldc) markers for astrocytes, in purified tdT+cells. (c) Immunocytochemistry confirming SOX2 expression in spinal astrocytes infected with thehGFAP-GFP-T2A-SOX2virus. (d) Confocal images showing astrocyte-derived neurons in the spinal cord transplanted with the SOX2 but not control virus-infected astrocytes. Orthogonal views of cells in the boxed regions are shown in the right panels. Astrocyte-derived neurons (tdT+TUBB3+or tdT+MAP2+) are indicated by arrows. Scale bars, 60 μm (b,c) and 30 μm (d). Figure 4: In vivo conversion of engrafted astrocytes to neurons. ( a ) Experimental scheme. Spinal astrocytes cultured from mGfap-Cre;Rosa-tdT mice were purified based on tdT expression. Three dpi, cells were infected with lentivirus and transplanted into the spinal cord of NSG mouse. ( b ) Immunocytochemistry showing the expression of GFAP and Aldolase c (Aldc) markers for astrocytes, in purified tdT + cells. ( c ) Immunocytochemistry confirming SOX2 expression in spinal astrocytes infected with the hGFAP-GFP-T2A-SOX2 virus. ( d ) Confocal images showing astrocyte-derived neurons in the spinal cord transplanted with the SOX2 but not control virus-infected astrocytes. Orthogonal views of cells in the boxed regions are shown in the right panels. Astrocyte-derived neurons (tdT + TUBB3 + or tdT + MAP2 + ) are indicated by arrows. Scale bars, 60 μm ( b , c ) and 30 μm ( d ). Full size image Cell proliferation during induced neurogenesis SOX2-induced neurons could be converted from astrocytes by a direct lineage switch without the addition of new cells. We tested this hypothesis by examining cell proliferation during the process of SOX2-induced neurogenesis. Proliferating cells in the injured adult spinal cord were continually labelled by intraperitoneal injection of 5-bromo-2'-deoxyuridine (BrdU) (100 mg kg −1 , twice a day) from 3–18 days post viral injection. When examined at 4 wpi, around 90% of induced DCX + cells were clearly labelled by BrdU indicating that they passed through a proliferative stage ( Fig. 5a,c ). Interestingly, nearly 17% of DCX + cells also expressed the cell proliferation marker Ki67, indicating that these cells were still in a cycling state ( Fig. 5b,c ). Using TUBB3 as an additional marker for neurons, we found that ~3% of neurons surrounding the core viral injection sites could be labelled by BrdU ( Fig. 5d,f ). Administration of BrdU during 4–8 wpi also led to a similar number of TUBB3 + cells being labelled ( Fig. 5e,f ). These data collectively demonstrate that adult neurogenesis induced by the ectopic expression of SOX2 is a continuous process, which passes through a proliferation phase. 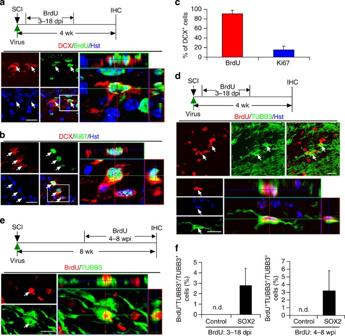Figure 5: Cell proliferation during SOX2-induced neurogenesis in the adult spinal cord. (a) Incorporation of BrdU in SOX2-induced DCX+cells. An orthogonal view of BrdU+DCX+cells in the boxed region is shown in the right panel (wk, weeks; IHC, immunohistochemistry). (b) Ki67-staining showing that SOX2-induced DCX+cells are proliferative at 5 wpi. An orthogonal view of Ki67+DCX+cells in the boxed region is shown in the right panel. (c) Quantification of BrdU or Ki67-labelled DCX+cells (mean+s.d.;n=3 mice per group). (d,e) Newly generated neurons indicated by BrdU-traced TUBB3+cells in the adult spinal cord. Orthogonal views of BrdU+TUBB3+cell are also shown. (f) Quantification of SOX2-induced new neurons (indicated by BrdU+TUBB3+) surrounding the virus-injected regions in adult spinal cords (mean+s.d.;n=3 mice per group; n.d., not detected). Scale bar, 20 μm (a,b,d,e). Figure 5: Cell proliferation during SOX2-induced neurogenesis in the adult spinal cord. ( a ) Incorporation of BrdU in SOX2-induced DCX + cells. An orthogonal view of BrdU + DCX + cells in the boxed region is shown in the right panel (wk, weeks; IHC, immunohistochemistry). ( b ) Ki67-staining showing that SOX2-induced DCX + cells are proliferative at 5 wpi. An orthogonal view of Ki67 + DCX + cells in the boxed region is shown in the right panel. ( c ) Quantification of BrdU or Ki67-labelled DCX + cells (mean+s.d. ; n =3 mice per group). ( d , e ) Newly generated neurons indicated by BrdU-traced TUBB3 + cells in the adult spinal cord. Orthogonal views of BrdU + TUBB3 + cell are also shown. ( f ) Quantification of SOX2-induced new neurons (indicated by BrdU + TUBB3 + ) surrounding the virus-injected regions in adult spinal cords (mean+s.d. ; n =3 mice per group; n.d., not detected). Scale bar, 20 μm ( a , b , d , e ). Full size image SOX2 induces neuroblasts in the adult spinal cord Ectopic expression of SOX2 alone was able to convert fibroblasts or human cortical astrocytes to proliferative and multipotent NSCs [28] , [38] , raising the possibility that spinal astrocytes could be similarly reprogrammed by SOX2. Spinal astrocytes were isolated from early postnatal mGfap-Cre;Rosa-tdT mice and infected with lentivirus expressing either GFP-T2A-SOX2 or the control GFP alone ( Fig. 6a,b ). Three days later, the fetal bovine serum-containing medium for astrocytes was switched to complete synthetic medium for NSCs. Neurospheres, which indicate the presence of self-renewable NSCs, were observed as early as 7 dpi in cultures with ectopic SOX2 but not the control GFP ( Fig. 6c,d ). These spheres were clearly labelled by tdT and GFP indicating an origin for SOX2 virus-infected astrocytes. Consistent with neural stem-like cells being present in postnatal spinal cords [39] , neurospheres were also detectable in the GFP group by 14 dpi. However, their number was significantly lower than that in the SOX2 group ( Fig. 6d ). Interestingly, ectopic SOX2 further dramatically enhanced the generation of secondary neurospheres from the primary ones ( Fig. 6c,d ). These spheres and the single cells dissociated from them were labelled by tdT, GFP and the NSC marker nestin (NES; Fig. 6e ). When cultured under differentiation conditions for 6 days, neurosphere-derived single cells could become TUBB3 + neurons, GFAP + astrocytes and NG2 + oligodendrocyte precursors ( Fig. 6f ). All of these cells were traced by the marker tdT indicating an origin from astrocytes. Together, these data show that SOX2 can promote the generation of multipotent NSCs from spinal astrocytes in culture consistent with results from cultured fibroblasts and cortical astrocytes [28] , [38] . 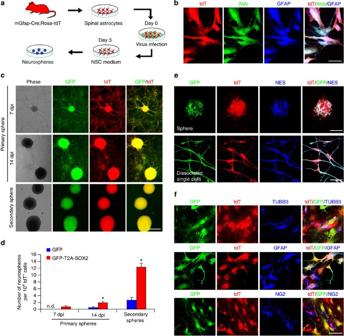Figure 6: Induction of NSCs from spinal astrocytes by SOX2 in culture. (a) Experimental scheme. (b) Immunocytochemistry confirming the astrocyte identity of cultured tdT+cells. (c) Representative micrographs of neurospheres from spinal astrocytes infected with thehGFAP-GFP-T2A-SOX2lentivirus. (d) Frequency of neurosphere-forming cells from spinal astrocytes infected with the indicated lentivirus. Secondary spheres were quantified at 7 days after plating (mean+s.d.;n=5; *P<0.01 by Student’st-test). (e) Nestin (NES) expression in SOX2-induced neurospheres. (f) Multiple lineage differentiation of SOX2-induced secondary neurospheres. Immunocytochemistry was performed 6 days after plating dissociated single cells. Scale bars, 50 μm (b), 200 μm (c), 60 μm (e) and 40 μm (f). Figure 6: Induction of NSCs from spinal astrocytes by SOX2 in culture. ( a ) Experimental scheme. ( b ) Immunocytochemistry confirming the astrocyte identity of cultured tdT + cells. ( c ) Representative micrographs of neurospheres from spinal astrocytes infected with the hGFAP-GFP-T2A-SOX2 lentivirus. ( d ) Frequency of neurosphere-forming cells from spinal astrocytes infected with the indicated lentivirus. Secondary spheres were quantified at 7 days after plating (mean+s.d. ; n =5; * P <0.01 by Student’s t -test). ( e ) Nestin (NES) expression in SOX2-induced neurospheres. ( f ) Multiple lineage differentiation of SOX2-induced secondary neurospheres. Immunocytochemistry was performed 6 days after plating dissociated single cells. Scale bars, 50 μm ( b ), 200 μm ( c ), 60 μm ( e ) and 40 μm ( f ). Full size image We then examined the SOX2-induced neurogenesis in the adult spinal cord using immunohistochemistry. A time course analysis showed that DCX + cells were not readily detectable until 4 wpi suggesting that the induced neurogenesis was a slow process. SSEA1 (also known as LeX or CD15) and KLF4, markers for multipotent stem cells, were not expressed in virus-infected astrocytes or the induced DCX + cells in the adult spinal cord at 1, 2, 3 or 4 wpi ( Fig. 7a ). Interestingly, SOX1 and SOX3, members of the SOXB1 subfamily of SOX transcription factors and key players in neural progenitors, were expressed in a subset of SOX2 virus-infected astrocytes, although these two factors were also distributed in some of the non-infected cells ( Fig. 7b ). The expression of SOX1 and SOX3 persisted into the DCX + stage, consistent with their reported expression in neuroblasts in the subventricular zone of the adult mouse brain [40] , [41] . 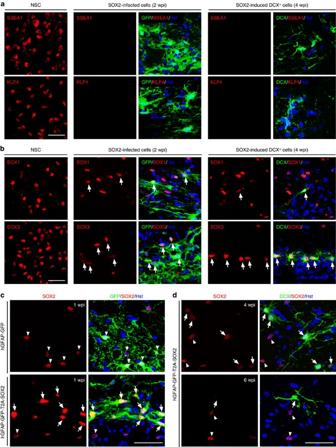Figure 7: Expression of SOXB1 factors during the reprogramming process. (a) Markers for multipotent stem cells are not detectable in the spinal cord injected with thehGFAP-GFP-T2A-SOX2virus. The expression in NSCs was served as a control. (b–d) The SOXB1 transcription factors are expressed during the reprogramming process. (b) Expression of SOX1 and SOX3 in SOX2 virus-infected cells and induced neuroblasts (indicated by arrows). Cultured NSCs served as controls. (c) Robust expression of SOX2 in the spinal cord injected with thehGFAP-GFP-T2A-SOX2virus (indicated by arrows). Arrowheads indicate endogenous SOX2 expression. (d) Downregulation of SOX2 in converted neuroblasts (indicated by arrows). Arrowheads indicate endogenous SOX2 expression. Scale bar, 40 μm (a–d). Figure 7: Expression of SOXB1 factors during the reprogramming process. ( a ) Markers for multipotent stem cells are not detectable in the spinal cord injected with the hGFAP-GFP-T2A-SOX2 virus. The expression in NSCs was served as a control. ( b – d ) The SOXB1 transcription factors are expressed during the reprogramming process. ( b ) Expression of SOX1 and SOX3 in SOX2 virus-infected cells and induced neuroblasts (indicated by arrows). Cultured NSCs served as controls. ( c ) Robust expression of SOX2 in the spinal cord injected with the hGFAP-GFP-T2A-SOX2 virus (indicated by arrows). Arrowheads indicate endogenous SOX2 expression. ( d ) Downregulation of SOX2 in converted neuroblasts (indicated by arrows). Arrowheads indicate endogenous SOX2 expression. Scale bar, 40 μm ( a – d ). Full size image Although endogenous SOX2 is broadly expressed in astrocytes in the adult spinal cord [42] , immunostaining showed that cells infected with the hGFAP-GFP-T2A-SOX2 virus had a significantly higher level of total SOX2 expression when compared with the surrounding non-infected cells ( Fig. 7c ). In induced DCX + cells, SOX2 expression was downregulated to a level similar to their neighbouring non-DCX + cells at 4 wpi and became almost non-detectable at 6 wpi ( Fig. 7d ). We hypothesized that such dynamic expression of SOX2 that was delivered by the hGFAP promoter was critical for induced neurogenesis. This hypothesis was tested by controlling SOX2 expression through the constitutively active CMV early enhancer/chicken beta actin ( CAG ) promoter. Robust SOX2 expression was observed in virus-infected cells; however, DCX + cells were not detected at 4 wpi ( Supplementary Fig. 7 ). These results suggest that the initial higher level of SOX2 expression and its subsequent downregulation was indeed necessary for the reprogramming process. In summary, these results reveal that the ectopic expression of SOX2 reprograms resident astrocytes to proliferative DCX + neuroblasts in the adult spinal cord contrary to in vitro cell culture conditions that enable SOX2 to convert astrocytes to multipotent stem cells ( Fig. 6 ). This highlights the importance of the cellular milieu on the reprogramming process. Induced neuroblasts mature into synapse-forming interneurons As DCX is restricted to neuroblasts and immature neurons and TUBB3 is also broadly expressed in both immature and mature neurons, the expression of these two markers during SOX2-induced neurogenesis does not indicate that these new neurons can become mature. In comparison, MAP2 and NeuN are markers for mature neurons. These markers were undetected in both BrdU- and tdT-traced cells in mGfap-Cre;Rosa-tdT mice that were injected with SOX2-expressing virus at 4 wpi ( Fig. 8a,f,g ). When examined at 8 wpi, however, ~3% of tdT + cells were labelled by either MAP2 or NeuN around the virus-injected region ( Fig. 8b,c,f ). Correspondingly, an estimated 1% of either MAP2- or NeuN-positive cells within the injected region also incorporated BrdU ( Fig. 8d,e,g ), indicating that they were mature neurons reprogrammed through cell division. VPA is a histone deacetylase inhibitor that enhances cellular reprogramming [43] and promotes normal neurogenesis and maturation of induced adult neuroblasts in the adult brain [29] , [44] . Here, we examined the effect of VPA on SOX2-induced neurogenesis in the adult spinal cord. Interestingly, 4 weeks of intraperitoneal injection of VPA (100 mg kg −1 , twice daily) resulted in nearly a twofold increase of tdT + cells being labelled by either MAP2 or NeuN in mGfap-Cre;Rosa-tdT mice ( Fig. 8f ). These neurons could survive up to 30 wpi, the longest time examined ( Supplementary Fig. 8 ). Quantification of BrdU-labelled cells also showed a threefold increase of newly generated MAP2 + or NeuN + mature neurons ( Fig. 8g ). Together, these data indicate that SOX2-induced neurons become mature by 8 wpi and can be further enhanced by treatment with VPA. 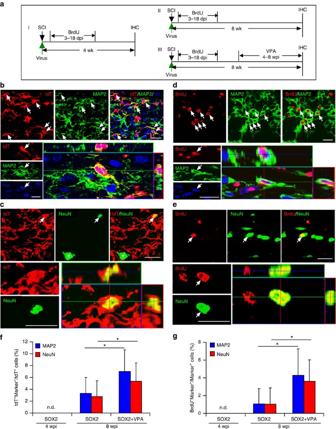Figure 8: Maturation of SOX2-induced new neurons in the injured adult spinal cord. (a) Experimental scheme.mGfap-Cre;Rosa-tdTmice were injected withhGFAP-SOX2or a control virus immediately after injury and analysed by IHC at 4 (I) or 8 (II, III) wpi. (b,c) Expression of the mature neuronal markers MAP2 (b) or NeuN (c) in tdT+cells in SOX2 virus-injected spinal cords at 8 wpi. tdT-traced MAP2+or NeuN+cells were not detectable in control virus-injected spinal cords. Orthogonal views of cells with expression of the indicated markers are also shown. Compared with endogenous spinal motoneurons (indicated by an asterisk inc), the SOX2-induced neurons are interneuron-like with a smaller soma (indicated by an arrow inc). (d,e) SOX2-induced mature neurons pass through a proliferative stage. Mice were treated with BrdU at 3–18 dpi and analysed at 8 wpi. Orthogonal views of BrdU-traced mature neurons are also shown. (f,g) Quantification of SOX2-induced mature neurons in the injured adult spinal cord (mean+s.d.;n=5 mice per group; *P<0.01 by Student’st-test). Scale bar, 20 μm (b–e). Figure 8: Maturation of SOX2-induced new neurons in the injured adult spinal cord. ( a ) Experimental scheme. mGfap-Cre;Rosa-tdT mice were injected with hGFAP-SOX2 or a control virus immediately after injury and analysed by IHC at 4 (I) or 8 (II, III) wpi. ( b , c ) Expression of the mature neuronal markers MAP2 ( b ) or NeuN ( c ) in tdT + cells in SOX2 virus-injected spinal cords at 8 wpi. tdT-traced MAP2 + or NeuN + cells were not detectable in control virus-injected spinal cords. Orthogonal views of cells with expression of the indicated markers are also shown. Compared with endogenous spinal motoneurons (indicated by an asterisk in c ), the SOX2-induced neurons are interneuron-like with a smaller soma (indicated by an arrow in c ). ( d , e ) SOX2-induced mature neurons pass through a proliferative stage. Mice were treated with BrdU at 3–18 dpi and analysed at 8 wpi. Orthogonal views of BrdU-traced mature neurons are also shown. ( f , g ) Quantification of SOX2-induced mature neurons in the injured adult spinal cord (mean+s.d. ; n =5 mice per group; * P <0.01 by Student’s t -test). Scale bar, 20 μm ( b – e ). Full size image We analysed the cellular identity of the reprogrammed neurons in mGfap-Cre;Rosa-tdT mice that were injected with hGFAP-SOX2 virus and treated with VPA for 4 weeks beginning at 4 wpi ( Fig. 9a ). These mice were also treated with BrdU from 3–18 dpi to label newly generated cells ( Fig. 9a ). Immunohistochemistry showed that none of the tdT + cells expressed choline acetyltransferase (ChAT), a marker for cholinergic motor neurons ( Supplementary Fig. 9a ). In contrast, the astrocyte-derived mature neurons (indicated by the expression of tdT and MAP2) were positive for GABA or vGLUT1, markers for inhibitory or excitatory neurons, respectively ( Fig. 9b and Supplementary Fig. 9b,c ). Importantly, co-staining with GABA and BrdU confirmed that these cells were indeed newly reprogrammed ( Fig. 9c ). The GABAergic neuronal identity was further demonstrated by staining with an antibody against glutamate decarboxylase (GAD65) ( Fig. 9d ). Interestingly, some tdT-traced cells were co-labelled by synapsin-1 (SYN1), a marker for presynaptic terminals, in spinal cords injected with SOX2 virus but not with a control virus ( Fig. 9e ). Confocal analyses under higher magnifications showed that dense bouton-like terminals co-stained with SYN1 and tdT were juxtaposed to the soma and axon of ChAT + cells ( Fig. 9f,g ), indicating the formation of synapses between SOX2-induced new neurons and local motor neurons. Together, these results showed that ectopic SOX2 could convert local astrocytes into synapse-forming GABAergic interneurons in the adult spinal cord. 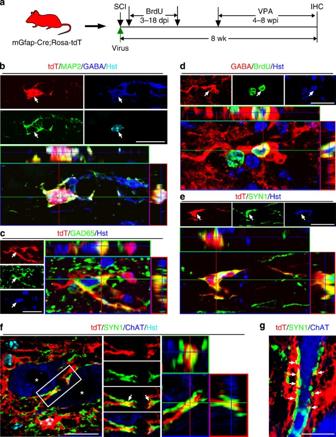Figure 9: SOX2-induced neurons resemble GABAergic interneurons in the adult spinal cord. (a) Experimental scheme to examine SOX2-induced mature neurons. (b,c) Ectopic SOX2 converts astrocytes (indicated by tdT) to GABAergic interneurons (indicated by GABA and GAD65 expression). Coexpression of the indicated markers is also shown by an orthogonal view. These cells were not detectable in spinal cords injected with a control virus. (d) BrdU labelling indicates that SOX2-induced GABA+cells are newly generated. Coexpression of the indicated markers is shown by an orthogonal view. (e) Expression of synapsin-I (SYN1) in tdT+cells in spinal cords injected with SOX2 but not a control virus. An orthogonal view is to show co-localization of the indicated markers. (f,g) Confocal images showing synapse-formation between SOX2-induced neurons (labelled by tdT) and the soma (f) or axon (g) of endogenous cholinergic motoneurons (labelled by ChAT). Synapses are indicated by SYN1-expression. Scale bar, 20 μm (b–f) and 10 μm (g). Figure 9: SOX2-induced neurons resemble GABAergic interneurons in the adult spinal cord. ( a ) Experimental scheme to examine SOX2-induced mature neurons. ( b , c ) Ectopic SOX2 converts astrocytes (indicated by tdT) to GABAergic interneurons (indicated by GABA and GAD65 expression). Coexpression of the indicated markers is also shown by an orthogonal view. These cells were not detectable in spinal cords injected with a control virus. ( d ) BrdU labelling indicates that SOX2-induced GABA + cells are newly generated. Coexpression of the indicated markers is shown by an orthogonal view. ( e ) Expression of synapsin-I (SYN1) in tdT + cells in spinal cords injected with SOX2 but not a control virus. An orthogonal view is to show co-localization of the indicated markers. ( f , g ) Confocal images showing synapse-formation between SOX2-induced neurons (labelled by tdT) and the soma ( f ) or axon ( g ) of endogenous cholinergic motoneurons (labelled by ChAT). Synapses are indicated by SYN1-expression. Scale bar, 20 μm ( b – f ) and 10 μm ( g ). Full size image Supporting the most recent results that the fate of non-neuronal cells in the adult brain could be reprogrammed in vivo [22] , [23] , [29] , [45] , we provide further evidence showing that the single transcription factor SOX2 is also sufficient to convert endogenous differentiated astrocytes into neuroblasts and mature neurons in the adult spinal cord with or without severe injury. The SOX2-induced neurogenesis passes through a proliferation phase and can give rise to synapse-forming interneurons. Postnatal spinal cords retain cells resembling NSCs that can self-renew and generate neurons, astrocytes and oligodendrocytes when cultured in vitro [39] , [46] . Although new neurons were reported in the adult spinal cord under physiological or pathological conditions [47] , [48] , the other studies rather showed that the adult spinal cord is not a neurogenic region and failed to identify new neurons under either the injured or uninjured state [4] , [6] , [49] , [50] . We are also unable to detect any newly generated neurons in the adult spinal cord non-injected or injected with lentivirus expressing the control GFP or other 11 transcription factors under the hGFAP promoter. Notwithstanding these discrepancies, spontaneous neurogenesis in the adult spinal cord is extremely limited, if there is any, and requires strategies to overcome this limitation. Through a combination of growth factor treatment and ectopic expression of the transcription factor NGN2, neurogenesis can be stimulated from endogenous proliferative neural progenitor cells in the adult spinal cord [50] . As an alternative strategy, our current study reveals that the fate of resident astrocytes can be reprogrammed to become neuroblasts and mature neurons in the adult spinal cord. NGN2-mediated differentiation of neural progenitors is a fast process with neurons being detectable as early as 3 days post injection, although a majority of the induced neurons cannot survive beyond 56 days even in the presence of exogenous BDNF [50] . In sharp contrast, our time course analyses reveal that SOX2-mediated in vivo reprogramming is a slow process with neuroblasts and mature neurons not readily detectable until 4 wpi and 8 wpi, respectively. Differentiated astrocytes might be more refractory to fate reprogramming as compared with neural progenitors [50] and thus potentially contribute to the slow reprogramming observed in our study. It is remarkable that SOX2-induced mature neurons from astrocytes were still detectable at 210 dpi when the mice were treated with VPA. Astrocytes are abundantly and ubiquitously distributed throughout the central nervous system. In response to injury, they are activated, proliferate and contribute to the formation of a glial scar [24] , [25] , [51] . These reactive astrocytes play a critical role in sealing the lesion site in the early phase of neural damage but constitute a mechanical and biochemical obstacle to axonal regeneration at later stages [52] . When isolated and cultured in vitro , activated astrocytes can form neurospheres that are able to generate neurons, oligodendrocytes and astrocytes [51] , [53] . Glutamatergic and GABAergic neurons can be, respectively, induced from reactive astrocytes by the forced expression of NGN2 and DLX2 in culture [27] . Despite these observations, astrocyte-derived neurons are not detectable around injured regions of the brain or spinal cord [4] , [6] , [49] , [50] , [51] , [54] . Nonetheless, these data indicate that endogenous astrocytes might be ideal targets for in vivo lineage reprogramming. Supporting this hypothesis, our in vivo screens for reprogramming factors and genetic lineage tracings showed that ectopic SOX2 uniquely converts resident astrocytes to DCX + neuroblasts and MAP2 + mature neurons in the adult spinal cord. NG2 + cells are also amenable to fate reprogramming [15] , [22] ; however, SOX2 under the hGFAP promoter is rarely expressed in these cells, potentially accounting for our failure to detect induced neuroblasts from these cells in the adult spinal cord. Reprogramming of somatic cells into neurons represents a novel approach towards understanding and treating neural injury and degeneration. The reprogramming process can be initiated by a few cell fate-determining transcription factors in culture [55] . SOX2, a high-mobility group DNA-binding domain transcription factor [56] , is essential for specification and/or maintenance of progenitor identity [57] , [58] , [59] . It also plays a key role in reprogramming somatic cells to pluripotent stem cells or NSCs in culture [8] , [38] , [60] , [61] , [62] , [63] . After screening pools of transcriptional regulators, we previously showed that SOX2 is alone sufficient to convert resident astrocytes to neuroblasts in the adult brain [29] . Nevertheless, it is not clear whether astrocytes in different regions of the central nervous system can be similarly reprogrammed, as they exhibit regional diversity [64] . It might not be coincident, though, that our additional screens also identified SOX2 as a key reprogramming factor in the adult spinal cord. Interestingly, SOX2 is endogenously expressed in spinal astrocytes [42] ; yet, no new neurons are detected in the spinal cord injected with the control virus or virus expressing many other transcription factors in our study. This suggests that a threshold of SOX2 expression is required to induce cell fate change. SOX2 expression under the hGFAP promoter is dynamic with a much higher level in reactive astrocytes and a subsequent downregulation in converted neuroblasts. The initial robust SOX2 expression may induce a ‘plastic’ state in infected astrocytes and cues in the local environment may help push them towards a neuroblast phenotype in vivo . A future detailed analysis is required to tease out the underlying molecular mechanism. Injury to spinal cords frequently disrupts the long ascending and descending spinal tracts and leads to functional impairments and long-term disability. There is currently no effective treatment for SCI. Reconstructing the neural circuits to mediate transmission of electrical impulses through the lesion site has been a major research focus [65] . Indeed, transplanted neurons are able to reinstate the disrupted neural circuitry in a mouse model of SCI [66] . Our present study demonstrates that SOX2-induced adult neurogenesis can generate mature neurons with features of GABAergic interneurons in injured VPA-treated spinal cords. The new neurons are capable of forming synapses with preexisting ChAT + motor neurons, suggesting potential integration into the local neural network of the injured spinal cord. Future work will examine whether induced neurons can form intraspinal relays that are able to mediate communication between segments above and below the lesion site. In summary, the results of this study raise a promising potential for treating SCI through cellular regeneration by in situ conversion of patients’ endogenous glial cells to neurons. This strategy might face fewer obstacles to clinical applications than other approaches since exogenous cells and transplantation are not required. However, the current reprogramming efficiency and the number of converted neurons are low. Further studies are necessary to enhance the reprogramming process and to define a precise strategy to generate subtype-specific neurons that are required for functional recovery after SCI. Animals Wild-type male C57/BL6J and the immunodeficient NSG mice were purchased from the Jackson Laboratories. The following transgenic mice have been previously described and were obtained from the Jackson Laboratories: mGfap-Cre line 77.6 (ref. 67 ), Ng2-Cre (ref. 36 ), Rosa-tdT [37] and Rosa-YFP [68] . Adult male and female mice at 2–3 months of age were used unless otherwise stated. All mice were housed under a 12 h light/dark cycle and had ad libitum access to food and water in the UT Southwestern animal facility. No statistical method was used to predetermine sample size. The experiments were not randomized and the experimenters were not blinded to the allocation of animals during experiments and outcome assessment. All experimental procedures and protocols were approved by the Institutional Animal Care and Use Committee at UT Southwestern. SCI model Surgeries were conducted under deep anaesthesia induced by a cocktail of ketamine and xylazine [69] . Briefly, a laminectomy was performed to expose the dorsal surface of the T7-9 segment. A hemisection was then introduced at the right side of the spinal cord by cutting twice at the same place using a fine corneal blade. After surgery, animals were returned to their home cages and received manual bladder expression twice daily until reflexive bladder control returned. Lentivirus preparation and stereotactic injection Lentivirus was used to deliver candidate factors into the adult spinal cords. Lentiviral vector hGFAP-GFP was generated by sub-cloning the synthetic hGFAP promoter [30] into CS-CDF-CG-PRE vector with EcoRI and AgeI sites. Candidate genes from human or mouse sources were then amplified by PCR and sub-cloned into the hGFAP-GFP vector by replacing the GFP gene at AgeI and XhoI sites. The third generation, replication-deficient lentivirus was generated in HEK293T cells by transient transfections with lentiviral vectors and the packaging plasmids (pMDL, VSV-G and pREV). Lentivirus was collected, precipitated with polyethylene glycol 8,000, and concentrated by centrifugation. Viral titres were determined by measuring the coexpressed GFP or antibody staining after infection of Cos-7 cells [70] . Using a Hamilton syringe and a 33 gauge, 45 degree-beveled needle (Hamilton, Reno, NV), 1.5 μl of lentivirus (0.5–2 × 10 9 colony-forming unit per ml) was manually injected into the spinal cord parenchyma at each of the two locations 3-mm apart at the T8 level. For animals with injured spinal cords, 1.5 μl of virus was immediately injected after hemisection at each of the two locations (1.5 mm proximal and distal to the lesion site). Virus was slowly injected within 1 min, followed by holding the needle at the injection site for 3 min and another minute to slowly withdraw the injection needle. BrdU labelling Proliferating cells in the spinal cord were labelled by intraperitoneal injection of BrdU (Sigma) at a dose of 100 mg kg −1 body weight, twice daily for the indicated duration. BrdU incorporation was detected by fluorescent staining using an anti-BrdU antibody (rat, 1:500, Accurate Chemical). Immunohistochemistry Mice were killed by CO 2 overdose and fixed by intracardial perfusion with 4% (w/v) paraformaldehyde in phosphate-buffered saline. Spinal cords were surgically dissected out, post-fixed overnight and cryoprotected with 30% sucrose at 4 °C for 48 h. Transverse sections or 1.5-cm longitudinal sections of spinal cords spanning the injection/injury sites were sectioned on a cryostat set at 14-μm thickness. The primary antibodies listed in Supplementary Table 1 were used for immunohistochemical analyses. Alexa Fluor 488-, 594- or 647-conjugated corresponding secondary antibodies from Jackson ImmunoResearch were used for indirect fluorescence. Nuclei were counterstained with Hoechst 33342 (Hst). Images were captured and examined by an Olympus fluorescence microscope or a Zeiss LSM 510 confocal microscope. A Cell Counter software plugin in the ImageJ programme was used for cell counting. Primary astrocyte culture Primary astrocytes were isolated from the spinal cord of postnatal day 2–4 mGfap-Cre;Rosa-tdT mouse. After removal of the meninges, the spinal cord was dissociated into a single-cell suspension through trypsinization and mechanical disruption. Cells were pelleted for 5 min at 1,000 r.p.m., re-suspended and plated in DMEM/F12 (1:1) medium containing 15% fetal bovine serum (Life Technologies). Culture medium was replaced 24 h later and every 3 days thereafter. When cultures became confluent, loosely attached microglia and oligodendrocyte precursor cells were removed from the cell monolayer by shaking vigorously. Cells were then passaged after dissociation with trypsin/EDTA. Neurosphere formation assays Spinal astrocytes from the mGfap-Cre;Rosa-tdT mice were purified through fluorescence-activated cell sorting based on tdT expression. These astrocytes were then infected with the hGFAP-GFP-T2A-SOX2 or hGFAP-GFP lentivirus. Three days later, the culture was switched to NSC medium, which consists of DMEM:F12:Neurobasal (2:2:1), 0.8% N2, 0.4% B27 (Life Technologies), 20 ng ml −1 FGF2 and 20 ng ml −1 EGF (Peprotech). Primary neurospheres were collected at day 14 and serially passaged under the same culture condition. To induce differentiation, secondary neurospheres were dissociated into single cells, which were then seeded onto Matrigel-coated glass coverslips in 24-well plate at a density of 2 × 10 4 cells per well. Cells were further cultured for 6 days in the NSC medium without FGF2 and EGF. Immunocytochemistry was performed on 4% paraformaldehyde-fixed cells using the indicated primary antibodies. Cell transplantation Purified tdT + spinal astrocytes were infected with the hGFAP-GFP-T2A-SOX2 or hGFAP-GFP lentivirus. Three days later, these cells (1 × 10 5 per 1.5 μl) were stereotactically injected into the spinal cord of 2–3 month old NSG mice at T7-9 segment using a pulled glass micropipette with an inner diameter of 40 μm. Animals were killed 4 or 5 weeks after transplantation. A 1.5-cm length of the spinal cord centred at the injection site was separated and subjected to immunohistochemical analyses. Statistical analysis The quantitative data were expressed as mean±s.d. from three to five mice. Statistical analysis was performed using unpaired Student’s t -tests. Differences were considered significant at P <0.05. How to cite this article: Su, Z. et al . In vivo conversion of astrocytes to neurons in the injured adult spinal cord. Nat. Commun. 5:3338 doi: 10.1038/ncomms4338 (2014).